LIF negatively regulates tumour-suppressor p53 through Stat3/ID1/MDM2 in colorectal cancers Leukaemia inhibitory factor (LIF) has been recently identified as a p53 target gene, which mediates the role of p53 in maternal implantation under normal physiological conditions. Here we report that LIF is a negative regulator of p53; LIF downregulates p53 protein levels and function in human colorectal cancer (CRC) cells. The downregulation of p53 by LIF is mediated by the activation of Stat3, which transcriptionally induces inhibitor of DNA-binding 1 ( ID1 ). ID1 upregulates MDM2, a key negative regulator of p53, and promotes p53 protein degradation. LIF is overexpressed in a large percentage of CRCs. LIF overexpression promotes cellular resistance towards chemotherapeutic agents in cultured CRC cells and colorectal xenograft tumours in a largely p53-dependent manner. Overexpression of LIF is associated with a poor prognosis in CRC patients. Taken together, LIF is a novel negative regulator of p53, overexpression of LIF is an important mechanism for the attenuation of p53, which promotes chemoresistance in CRCs. p53 plays a critical role in tumour suppression [1] , [2] . p53 is the most frequently mutated gene in human cancers; over 50% of all cancers harbour p53 mutations [3] . As a transcription factor, p53 responds to stress signals and regulates the expression of its target genes, which leads to various cellular responses to prevent tumour formation [1] . As a haplo-insufficient gene, a little decrease in p53 levels or activities (for example, twofold difference) impacts greatly upon tumorigenesis [4] , [5] , [6] . p53 is under tight regulation by a number of negative regulators, including MDM2, MDM4, Wip1, Pirh2 and Cyclin G1, to maintain its proper activities and function in cells [7] , [8] , [9] . Many p53-negative regulators (for example, MDM2, Wip1, Pirh2 and Cyclin G1) are p53 target genes, which form autoregulatory-negative feedback loops with p53. Overexpression and/or amplification of these negative regulators have been frequently observed in tumours, which leads to the attenuation of p53 function and promotes tumorigenesis [10] , [11] . Colorectal cancer (CRC) is the third most commonly diagnosed cancer and the third leading cancer death in the United States [12] . Around 50% of CRCs contain p53 mutations. Loss of p53 function plays a critical role in colorectal tumorigenesis by driving the progression of adenoma to carcinoma [13] , [14] . p53 is also critical for chemotherapeutic response in CRCs. Loss of p53 abolishes the apoptotic response to 5-fluorouracil (5-FU), a most commonly used chemotherapeutic agent for CRCs, in both cultured CRC cells and animal models [15] , [16] . Clinical studies show that human CRCs with wild-type p53 display a better response to 5-FU-based chemotherapy compared with CRCs with p53 mutations [17] , [18] . These findings demonstrate a critical role of p53 in tumour suppression and chemotherapeutic response in CRCs. As a multi-functional protein, LIF plays different roles in a highly context-dependent manner. For instance, LIF induces the differentiation of murine myeloid leukaemia cells, whereas inhibits the differentiation of murine embryonic stem cells [19] , [20] . LIF also plays a crucial role in embryonic implantation [21] . LIF functions in autocrine and/or paracrine manners through binding to the LIF receptor complex composed of the LIF receptor and gp-130, which in turn activates selective pathways, including the PI3K/AKT and JAK/Stat3 pathways, depending on the context [22] , [23] , [24] . Recently, we identified LIF as a novel p53 target gene. LIF is an important component of the p53 pathway, which mediates p53’s role in embryonic implantation [25] , [26] , [27] , [28] . Considering the critical role of the p53 pathway in cancer, our findings suggest a potential role of LIF in cancer. However, to date, the role of LIF in tumorigenesis, especially CRC, is poorly understood. Here we report that LIF has an important role in regulation of p53 function in tumour suppression; LIF negatively regulates p53 protein levels and function in human CRC cells. The negative regulation of p53 by LIF is through the activation of Stat3, which in turn induces the expression of inhibitor of DNA-binding 1 (ID1), the helix–loop–helix (HLH) protein inhibitor of differentiation and DNA binding. ID1 upregulates MDM2 expression, which leads to accelerated p53 protein degradation. LIF is overexpressed in a large percentage of human CRCs and is associated with a poor prognosis of CRC patients. Overexpression of LIF promotes chemoresistance in both cultured CRC cells and colorectal xenograft tumours in a largely p53-dependent manner. Overexpression of LIF in human CRCs To study the potential role of LIF in CRCs, the expression of LIF was determined at both mRNA and protein levels in human CRC samples. The LIF mRNA levels were determined in 24 pairs of cDNA prepared from human CRC and their matched adjacent non-tumour tissues (Colorectal Cancer cDNA Array, Origene) by Taqman real-time PCR. LIF mRNA levels were significantly higher in CRCs than their adjacent non-tumour tissues (4.37-fold higher in average, P =6.6E−5; Fig. 1a ). Furthermore, LIF protein levels were determined in 25 pairs of formalin-fixed and paraffin-embedded CRC specimen and their matched adjacent non-tumour tissues by immunohistochemistry (IHC) staining. Consistently, a significantly higher percentage of CRC samples showed positive LIF staining (>10% cells are positively stained) compared with their matched adjacent non-tumour tissues (72% versus 20%, P =0.005; Fig. 1b ). These results demonstrated that LIF is overexpressed in a high percentage of CRCs, which suggests a potential role of LIF overexpression in colorectal tumorigenesis. 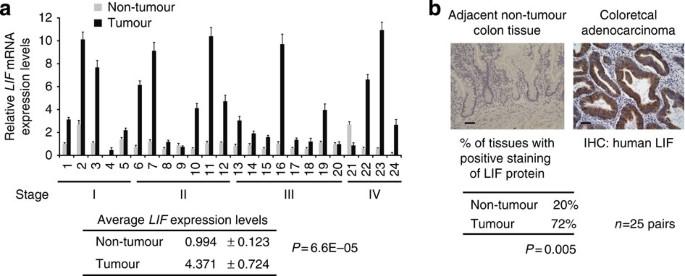Figure 1: Overexpression of LIF in human CRCs. (a) Human CRC tissues display significantly higherLIFmRNA expression levels compared with adjacent non-tumour tissues. cDNAs prepared from human CRC samples and their matched adjacent non-tumour tissues were provided by Origene.LIFmRNA expression levels were measured by Taqman real-time PCR and normalized with actin.LIFexpression levels in a non-tumour tissue (#1) were designated as 1. Data were presented as mean±s.d. (n=3).Pvalue was obtained by Student’st-tests. (b) Higher LIF protein levels in human CRC tissues. LIF protein levels were determined by IHC in human CRC samples and their matched adjacent non-tumour tissues (n=25).P-value was obtained by Student’st-tests. Representative IHC staining results for LIF in CRCs (positive staining, right panel) and adjacent non-tumour colorectal tissues (negative staining, left panel) are shown. Positive LIF staining: >10% cells positively stained with LIF. Scale bar, 50 μm. Figure 1: Overexpression of LIF in human CRCs. ( a ) Human CRC tissues display significantly higher LIF mRNA expression levels compared with adjacent non-tumour tissues. cDNAs prepared from human CRC samples and their matched adjacent non-tumour tissues were provided by Origene. LIF mRNA expression levels were measured by Taqman real-time PCR and normalized with actin. LIF expression levels in a non-tumour tissue (#1) were designated as 1. Data were presented as mean±s.d. ( n =3). P value was obtained by Student’s t -tests. ( b ) Higher LIF protein levels in human CRC tissues. LIF protein levels were determined by IHC in human CRC samples and their matched adjacent non-tumour tissues ( n =25). P -value was obtained by Student’s t -tests. Representative IHC staining results for LIF in CRCs (positive staining, right panel) and adjacent non-tumour colorectal tissues (negative staining, left panel) are shown. Positive LIF staining: >10% cells positively stained with LIF. Scale bar, 50 μm. Full size image LIF inhibits p53-mediaetd chemoresponse in human CRC cells To investigate the potential role of LIF in CRCs, the effect of LIF on the cellular response towards chemotherapeutic agents was determined in a panel of human CRC cells. It has been well-established that p53 plays a central role in tumour suppression and is critical for an effective chemotherapeutic response in CRCs through induction of apoptosis. To this end, three pairs of isogenic human CRC cells with and without wild-type p53, including HCT116 p53 +/+ and p53 −/− , RKO p53 +/+ and p53 −/− , DLD-1 p53 +/+ and p53 −/− cells, were employed to establish stable cell lines with ectopic LIF expression. These cell lines were stably transduced with retroviral LIF expression vectors (pLPCX-LIF) (HCT116 p53 +/+ -LIF, HCT116 p53 −/− -LIF, RKO p53 +/+ -LIF, RKO p53 −/− -LIF, DLD-1 p53 +/+ -LIF and DLD-1 p53 −/− -LIF). Cells transduced with empty vectors served as controls. The ectopic LIF expression in cells was confirmed at the protein level by western blot assays ( Fig. 2a for HCT116 and RKO cells and Supplementary Fig. 1a for DLD-1 cells). The secretion of LIF into the conditioned medium (CM) was also confirmed ( Fig. 2a ). 5-FU clearly induced cell death in p53 +/+ human CRC cells (HCT116 p53 +/+ , RKO p53 +/+ and DLD-1 p53 +/+ ), whereas had a very limited effect on cell death in their isogenic p53 −/− cells. Notably, ectopic LIF expression markedly reduced 5-FU-induced cell death in p53 +/+ CRC cells, but showed no apparent effect in isogenic p53 −/− cells ( Fig. 2b for HCT116 and RKO cells, and Supplementary Fig. 1b for DLD-1 cells). A similar inhibitory effect of LIF on chemotherapeutic agents-induced cell death was observed in HCT116 p53 +/+ cells treated with etoposide (ETO) or adriamycin (ADR), but not in HCT116 p53 −/− cells that underwent same treatments ( Fig. 2c ). It has been well-established that 5-FU induces cell death in CRC cells mainly through p53-mediated apoptosis [15] . The effect of LIF on 5-FU-induced apoptosis was determined in above-mentioned cells by employing Annexin V staining. 5-FU induced apoptosis in a highly p53-dependent manner since very limited apoptosis was observed in p53 −/− cells treated with 5-FU ( Fig. 2d ), which is consistent with a previous report [15] . Notably, ectopic LIF expression markedly decreased 5-FU-induced apoptosis in p53 +/+ CRC cells ( Fig. 2d for HCT116 and RKO cells, and Supplementary Fig. 1c for DLD-1 cells). The inhibitory effect of LIF on p53-mediated apoptosis was further clearly demonstrated by the inhibition of activation and cleavage of caspase 3 and the subsequent proteolytic cleavage of poly (ADP ribose) polymerases (PARPs) by LIF in p53 +/+ but not p53 −/− CRC cells treated with 5-FU ( Fig. 2e for HCT116 and RKO cells, and Supplementary Fig. 1d for DLD-1 cells). The inhibitory effect of LIF on p53-mediated apoptosis was also observed in HCT116 p53 +/+ but not in HCT116 p53 −/− cells treated with ETO or ADR as determined by Annexin V staining and the levels of cleaved caspase 3 and PARP ( Supplementary Fig. 2a,b ). Knockdown of ectopic LIF in HCT116 p53 +/+ -LIF cells by short interfering RNA (siRNA) oligos blocked the inhibitory effect of LIF on 5-FU-induced apoptosis ( Fig. 2f ). Consistently, knockdown of endogenous LIF by siRNA in HCT116 p53 +/+ cells also clearly increased 5-FU-induced apoptosis ( Fig. 2g ). The knockdown of endogenous LIF was confirmed at both mRNA and protein levels ( Supplementary Fig. 3 ). Taken together, these results demonstrated that LIF inhibits p53-mediated apoptosis, which in turn promotes chemoresistance in CRC cells. 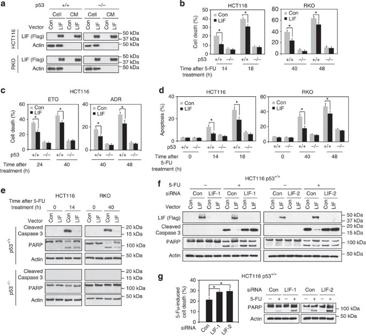Figure 2: LIF inhibits p53-mediated apoptosis in response to the treatments of chemotherapeutic agents in human CRC cells. (a) Two pairs of p53+/+and p53−/−human CRC cell lines with stable ectopic LIF expression (HCT116 p53+/+-LIF, HCT116 p53−/−-LIF, RKO p53+/+-LIF and RKO p53−/−-LIF cells) and their control cells were established by transduction of LIF expression vectors (pLPCX-LIF) and control vectors, respectively. Ectopic LIF expression in cells was detected by western blot assays. The secretion of LIF from cells into the conditioned medium (CM) was also detected by western blot assays. CM was collected after serum-free medium was cultured overnight with one-third number of the cells used for western blot assays. (b) LIF reduced 5-FU-induced cell death in a p53-dependent manner in cells. Above-mentioned cells with stable ectopic LIF expression and their control cells were treated with 5-FU (500 μM) for the indicated time periods. Cell viability was measured by the Vi-CELL cell counter. (c) LIF reduced etoposide (ETO)- and adriamycin (ADR)-induced cell death in a p53-dependent manner in HCT116 cells. HCT116 p53+/+-LIF, HCT116 p53−/−-LIF and their control cells were treated with ETO (30 μM) or ADR (5 μM) for the indicated time periods. (d,e) LIF reduced p53-meidated apoptosis induced by 5-FU in HCT116 and RKO cells. (d) The percentage of apoptotic cells was determined by Annexin V staining. (e) The levels of cleaved caspase 3 and PARP were determined by western blot assays. (f) Knockdown of LIF in HCT116 p53+/+-LIF cells by two different siRNA oligos largely abolished the inhibitory effect of LIF on 5-FU-induced apoptosis. 5-FU-induced apoptosis was determined by measuring the levels of cleaved caspase 3 and PARP. (g) Knockdown of endogenous LIF in HCT116 p53+/+cells increased 5-FU-induced apoptosis. Cell viability (left panel) and apoptosis (right panel) were determined by the Vi-CELL cell counter and the levels of cleaved PARP, respectively. Forb–d,g, data are presented as mean±s.d. (n=3). *P<0.001 (Student’st-test). Figure 2: LIF inhibits p53-mediated apoptosis in response to the treatments of chemotherapeutic agents in human CRC cells. ( a ) Two pairs of p53 +/+ and p53 −/− human CRC cell lines with stable ectopic LIF expression (HCT116 p53 +/+ -LIF, HCT116 p53 −/− -LIF, RKO p53 +/+ -LIF and RKO p53 −/− -LIF cells) and their control cells were established by transduction of LIF expression vectors (pLPCX-LIF) and control vectors, respectively. Ectopic LIF expression in cells was detected by western blot assays. The secretion of LIF from cells into the conditioned medium (CM) was also detected by western blot assays. CM was collected after serum-free medium was cultured overnight with one-third number of the cells used for western blot assays. ( b ) LIF reduced 5-FU-induced cell death in a p53-dependent manner in cells. Above-mentioned cells with stable ectopic LIF expression and their control cells were treated with 5-FU (500 μM) for the indicated time periods. Cell viability was measured by the Vi-CELL cell counter. ( c ) LIF reduced etoposide (ETO)- and adriamycin (ADR)-induced cell death in a p53-dependent manner in HCT116 cells. HCT116 p53 +/+ -LIF, HCT116 p53 −/− -LIF and their control cells were treated with ETO (30 μM) or ADR (5 μM) for the indicated time periods. ( d , e ) LIF reduced p53-meidated apoptosis induced by 5-FU in HCT116 and RKO cells. ( d ) The percentage of apoptotic cells was determined by Annexin V staining. ( e ) The levels of cleaved caspase 3 and PARP were determined by western blot assays. ( f ) Knockdown of LIF in HCT116 p53 +/+ -LIF cells by two different siRNA oligos largely abolished the inhibitory effect of LIF on 5-FU-induced apoptosis. 5-FU-induced apoptosis was determined by measuring the levels of cleaved caspase 3 and PARP. ( g ) Knockdown of endogenous LIF in HCT116 p53 +/+ cells increased 5-FU-induced apoptosis. Cell viability (left panel) and apoptosis (right panel) were determined by the Vi-CELL cell counter and the levels of cleaved PARP, respectively. For b – d , g , data are presented as mean±s.d. ( n =3). * P <0.001 (Student’s t -test). Full size image LIF decreases p53 protein levels and function in CRC cells It has been well-established that in response to chemotherapeutic agents, including 5-FU, p53 is activated and its protein levels increase, which in turn initiates cellular responses, including apoptosis, to promote an efficient chemotherapeutic response [29] . The levels of p53 protein are one of the most important determinants of its functions, including apoptosis. As shown in Supplementary Fig. 4 , the degree of p53-meidated apoptosis is dependent upon the levels of p53 protein in H1299-Tet-on-p53 cells, which express p53 protein under the control of a doxycycline-regulated promoter. Whereas the cells did not express p53 protein in the absence of doxycycline, low concentrations of doxycycline (2.5, 50 ng ml −1 ) induced p53 protein at a low level, and high concentrations of doxycycline (1,000 ng ml −1 ) induced p53 protein at a much higher level. Furthermore, the levels of p53-mediated apoptosis were much lower in cells with low p53 protein levels than in cells with higher p53 levels ( Supplementary Fig. 4 ). The observation that LIF inhibits chemotherapeutic agent-induced apoptosis in a largely p53-dependent manner raised the possibility that LIF may negatively regulate p53 protein levels and function. To test this possibility, HCT116 p53 +/+ -LIF, RKO p53 +/+ -LIF, DLD-1 p53 +/+ -LIF and their control cells were treated with 5-FU. Their isogenic p53 −/− cells with and without ectopic LIF expression were also employed. The phosphorylation of p53 at Ser15 (p-p53), which is the initial step of p53 activation in response to 5-FU treatment, and the accumulation of p53 and p21 proteins, a well-known p53 target, were measured by western blot assays. The induction of p-p53, p53 and p21 proteins in response to 5-FU was significantly lower in cells with ectopic LIF expression compared with control cells ( Fig. 3a for HCT116 and RKO cells, and Supplementary Fig. 5a for DLD-1 cells). The inhibitory effect of LIF on 5-FU-induced p53 protein accumulation was observed in the majority of cells as determined in HCT116 p53 +/+ cells by immunofluorescence (IF) staining assays ( Supplementary Fig. 5b ). The inhibitory effect of LIF on 5-FU-induced p53 protein accumulation was also observed in non-apoptotic HCT116 p53 +/+ cells that were sorted as cells negative for Annexin V staining by using a cell sorter ( Supplementary Fig. 5c ). These results demonstrated that the inhibitory effect of LIF on p53 existed in a major population of cells. Similar results were observed in HCT116 p53 +/+ -LIF and control cells treated with ETO and ADR ( Fig. 3b ). LIF is a cytokine. The effect of exogenous LIF on p53 was also investigated. Exogenous LIF protein, which was used to treat cells directly, showed a similar inhibitory effect on the activation and accumulation of p53 protein, as well as the increase of p21 protein levels in response to 5-FU in HCT116 p53 +/+ and RKO p53 +/+ cells ( Supplementary Fig. 5d ). 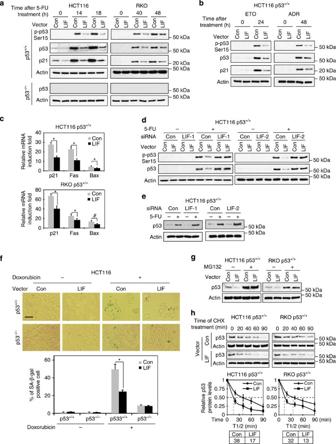Figure 3: LIF downregulates p53 protein levels and transcriptional activity through accelerating p53 protein degradation. (a) HCT116 p53+/+-LIF, HCT116 p53−/−-LIF, RKO p53+/+-LIF, RKO p53−/−-LIF and their control cells were treated with 5-FU. The levels of phosphorylated p53 at serine 15 (p-p53-Ser15), total p53 and p21 proteins were examined by western blot assays. (b) HCT116 p53+/+-LIF and its control cells were treated with ETO (30 μM) or ADR (5 μM). The levels of p-p53-Ser15, p53 and p21 proteins were examined by western blot assays. (c) HCT116 p53+/+-LIF, RKO p53+/+-LIF and their control cells were treated with 5-FU (500 μM), the mRNA levels ofp21,FasandBaxwere determined by Taqman real-time PCR and normalized withactin. (d) Knockdown of LIF in HCT116 p53+/+-LIF cells largely blocked the inhibitory effect of LIF on the activation and accumulation of p53 protein in response to 5-FU treatment (500 μM). (e) Knockdown of endogenous LIF in HCT116 p53+/+cells increased p53 protein levels in response to 5-FU treatment. (f) LIF negatively regulated p53 function in senescence. HCT116 p53+/+-LIF, HCT116 p53−/−-LIF and their control cells were treated with doxorubicin (50 nM) for 3 days before senescent cells were detected by senescence-associated β-galactosidase (SA-β-gal) staining. Upper panels: represented images of SA-β-gal staining of senescent cells. Scale bar, 100 μm. Lower panel: the percentage of SA-β-gal-positive cells. (g) Blocking proteasomal degradation by MG132 largely abolished the inhibitory effect of LIF on p53 protein levels in HCT116 p53+/+and RKO p53+/+cells. HCT116 p53+/+-LIF, RKO p53+/+-LIF and their control cells were treated with MG132 (30 μM) for 6 h. (h) LIF decreased p53 protein half-life. HCT116 p53+/+-LIF, RKO p53+/+-LIF and their control cells were treated with cycloheximide (CHX, 10 μg ml−1) for the indicated time before being collected for western blot analysis. Forc,f,h, data are presented as mean±s.d. (n=3). *P<0.001 (Student’st-test). Figure 3: LIF downregulates p53 protein levels and transcriptional activity through accelerating p53 protein degradation. ( a ) HCT116 p53 +/+ -LIF, HCT116 p53 −/− -LIF, RKO p53 +/+ -LIF, RKO p53 −/− -LIF and their control cells were treated with 5-FU. The levels of phosphorylated p53 at serine 15 (p-p53-Ser15), total p53 and p21 proteins were examined by western blot assays. ( b ) HCT116 p53 +/+ -LIF and its control cells were treated with ETO (30 μM) or ADR (5 μM). The levels of p-p53-Ser15, p53 and p21 proteins were examined by western blot assays. ( c ) HCT116 p53 +/+ -LIF, RKO p53 +/+ -LIF and their control cells were treated with 5-FU (500 μM), the mRNA levels of p21 , Fas and Bax were determined by Taqman real-time PCR and normalized with actin . ( d ) Knockdown of LIF in HCT116 p53 +/+ -LIF cells largely blocked the inhibitory effect of LIF on the activation and accumulation of p53 protein in response to 5-FU treatment (500 μM). ( e ) Knockdown of endogenous LIF in HCT116 p53 +/+ cells increased p53 protein levels in response to 5-FU treatment. ( f ) LIF negatively regulated p53 function in senescence. HCT116 p53 +/+ -LIF, HCT116 p53 −/− -LIF and their control cells were treated with doxorubicin (50 nM) for 3 days before senescent cells were detected by senescence-associated β-galactosidase (SA-β-gal) staining. Upper panels: represented images of SA-β-gal staining of senescent cells. Scale bar, 100 μm. Lower panel: the percentage of SA-β-gal-positive cells. ( g ) Blocking proteasomal degradation by MG132 largely abolished the inhibitory effect of LIF on p53 protein levels in HCT116 p53 +/+ and RKO p53 +/+ cells. HCT116 p53 +/+ -LIF, RKO p53 +/+ -LIF and their control cells were treated with MG132 (30 μM) for 6 h. ( h ) LIF decreased p53 protein half-life. HCT116 p53 +/+ -LIF, RKO p53 +/+ -LIF and their control cells were treated with cycloheximide (CHX, 10 μg ml −1 ) for the indicated time before being collected for western blot analysis. For c , f , h , data are presented as mean±s.d. ( n =3). * P <0.001 (Student’s t -test). Full size image p53 functions as a transcription factor. The effect of LIF on p53 function in transcriptional activity was determined in HCT116 p53 +/+ -LIF, RKO p53 +/+ -LIF, DLD-1 p53 +/+ -LIF and their control cells. The mRNA levels of a group of well-known p53 target genes, including p21 (involved in cell cycle arrest), Fas and Bax (involved in apoptosis), were examined before and after 5-FU treatment by Taqman real-time PCR. 5-FU clearly induced the transcription of all these genes. Notably, the induction of these genes was significantly lower in cells with ectopic LIF expression compared with that in control cells ( Fig. 3c for HCT116 p53 +/+ and RKO p53 +/+ cells, and Supplementary Fig. 5e for DLD-1 p53 +/+ cells). Knockdown of ectopic LIF by siRNA in HCT116 p53 +/+ -LIF cells largely abolished the inhibitory effect of LIF on 5-FU-induced activation and accumulation of p53 protein ( Fig. 3d ). Furthermore, knockdown of endogenous LIF clearly increased 5-FU-induced p53 protein accumulation in HCT116 p53 +/+ cells ( Fig. 3e ). The effect of LIF on p53 function in senescence was also determined in HCT116 p53 +/+ -LIF, HCT116 p53 −/− -LIF and their control cells. Cells were treated with doxorubicin, and senescent cells were detected by senescence-associated β-galactosidase assays. Doxorubicin effectively induced senescence in HCT116 cells in a largely p53-dependent manner ( Fig. 3f ). Notably, ectopic LIF expression clearly reduced doxorubicin-induced senescence in HCT116 p53 +/+ but not p53 −/− cells ( Fig. 3f ). p53 is mainly regulated at the post-translational level, and has a short protein half-life in cells under non-stressed conditions. Ectopic LIF expression did not clearly change p53 mRNA levels as determined by Taqman real-time PCR ( Supplementary Fig. 6 ). p53 protein is mostly turned over through proteasomal degradation. Blocking proteasomal degradation by MG132, a proteasomal inhibitor, clearly increased p53 protein levels in HCT116 p53 +/+ and RKO p53 +/+ cells. Importantly, MG132 treatment largely abolished the inhibitory effect of LIF on the p53 protein level in both cell lines ( Fig. 3g ). Consistently, the half-life of p53 protein was clearly decreased in HCT116 p53 +/+ -LIF and RKO p53 +/+ -LIF cells ( Fig. 3h ). Taken together, these results strongly suggest that LIF downregulates p53 protein levels and function through accelerating p53 protein degradation in cells. LIF upregulates MDM2 to downregulate p53 through Stat3 MDM2 is a key negative regulator of p53. As an E3 ubiquitin ligase, MDM2 binds to and ubiquitinates p53 for proteasomal degradation. Interestingly, we found that LIF increased the expression of MDM2 at both mRNA and protein levels ( Fig. 4a ). Knockdown of MDM2 in HCT116 p53 +/+ -LIF cells by siRNA oligos blocked the inhibitory effect of LIF on p53 protein accumulation in response to 5-FU treatment ( Fig. 4b ). Stat3 is a critical downstream effector of the LIF signalling in many types of cells and tissues [19] , [23] . To investigate whether the activation of Stat3 by LIF mediates the inhibitory effect of LIF on p53 protein levels and function in CRC cells, Stattic, a specific Stat3 inhibitor, was employed to block Stat3, and the effect of LIF on p53 was determined. HCT116 p53 +/+ -LIF, RKO p53 +/+ -LIF and their control cells were treated with 5-FU along with or without Stattic treatment. Stattic greatly attenuated the inhibitory effect of LIF on 5-FU-induced cell death as well as the p53-mediated apoptosis induced by 5-FU ( Fig. 4c,d ). Importantly, Stattic treatment largely abolished the inhibitory effect of LIF on 5-FU-induced activation and accumulation of p53 protein in HCT116 p53 +/+ and RKO p53 +/+ cells ( Fig. 4d ). Stattic treatment also largely abolished the inhibitory effect of LIF on p53 transcriptional activity towards its target genes, including p21 and Fas , in HCT116 p53 +/+ cells ( Fig. 4e ). Consistent results were obtained when the Stat3 function was blocked by using siRNA targeting Stat3. Knockdown of endogenous Stat3 by siRNA largely abolished the inhibitory effect of LIF on 5-FU-induced apoptosis, the activation and accumulation of p53 protein in HCT116 p53 +/+ cells ( Fig. 4f and Supplementary Fig. 7a ). Importantly, the upregulation of MDM2 levels by LIF is largely mediated by Stat3; Stattic clearly blocked the increase of MDM2 levels in HCT116 p53 +/+ -LIF and RKO p53 +/+ -LIF cells ( Fig. 4g ). Consistently, ectopic Stat3 expression in HCT116 p53 +/+ cells clearly increased MDM2 mRNA and protein levels ( Fig. 4h ). Although Stat3 expression did not have an apparent effect on p53 mRNA levels ( Supplementary Fig. 7b ), it clearly decreased the activation and accumulation of p53 protein in response to 5-FU treatment ( Fig. 4i ). Collectively, these results demonstrated that LIF activates the Stat3 signalling pathway, which in turn upregulates MDM2 and downregulates p53 protein levels and function. 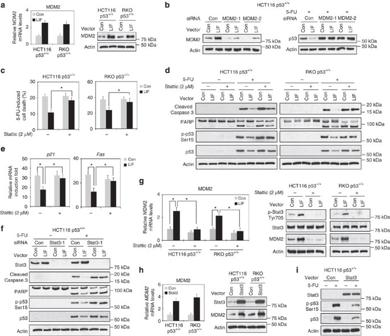Figure 4: LIF upregulates MDM2 to downregulate p53 through activation of the Stat3 signalling. (a) LIF increased the expression levels of MDM2. The mRNA and protein levels of MDM2 were examined in HCT116 p53+/+-LIF, RKO p53+/+-LIF and their control cells. (b) Knockdown of MDM2 in HCT116 p53+/+-LIF cells largely blocked the inhibitory effect of LIF on 5-FU-induced p53 protein accumulation (right panel). The knockdown of MDM2 was confirmed at the protein levels (left panel). (c,d) HCT116 p53+/+-LIF, RKO p53+/+-LIF and their control cells were treated with 5-FU (500 μM) along with or without Stattic (2 μM), a specific inhibitor of Stat3. (c) Cell viability was measured by Vi-CELL cell counter. (d) The levels of cleaved caspase 3, PARP, p-p53-Ser15 and p53 proteins were examined by western blot assays. (e) HCT116 p53+/+-LIF and its control cells were treated with 5-FU along with or without Stattic. The mRNA levels ofp21andFaswere determined by Taqman real-time PCR and normalized withactin. (f) HCT116 p53+/+-LIF and its control cells were transfected with siRNA targeting Stat3 (siRNA Stat3-1) or control siRNA, followed by 5-FU treatment. The levels of Stat3, cleaved caspase 3, PARP, p-p53-Ser15 and p53 proteins were determined by western blot assays. Similar results were obtained when a different Stat3 siRNA (siRNA Stat3-2) were used (seeSupplementary Fig. 7a). (g) The upregulation of MDM2 by LIF was largely abolished by Stattic. HCT116 p53+/+-LIF, RKO p53+/+-LIF and their control cells were treated with Stattic. TheMDM2mRNA levels were determined by Taqman real-time PCR and normalized withactin(left panel). The levels of phosphorylated Stat3 at Tyrosine 705 (p-Stat3-Tyr705), Stat3 and MDM2 proteins were examined by western blot assays (right panels). (h) Stat3 increased the expression levels of MDM2. The MDM2 mRNA and protein levels were examined in HCT116 p53+/+and RKO p53+/+cells transfected with Stat3 expression vectors or control vectors. (i) Ectopic Stat3 expression reduced the activation and accumulation of p53 protein in response to 5-FU in HCT116 p53+/+cells. Fora,c,e,g,h, data are presented as mean±s.d. (n=3). *P<0.001 (Student’st-test). Figure 4: LIF upregulates MDM2 to downregulate p53 through activation of the Stat3 signalling. ( a ) LIF increased the expression levels of MDM2. The mRNA and protein levels of MDM2 were examined in HCT116 p53 +/+ -LIF, RKO p53 +/+ -LIF and their control cells. ( b ) Knockdown of MDM2 in HCT116 p53 +/+ -LIF cells largely blocked the inhibitory effect of LIF on 5-FU-induced p53 protein accumulation (right panel). The knockdown of MDM2 was confirmed at the protein levels (left panel). ( c , d ) HCT116 p53 +/+ -LIF, RKO p53 +/+ -LIF and their control cells were treated with 5-FU (500 μM) along with or without Stattic (2 μM), a specific inhibitor of Stat3. ( c ) Cell viability was measured by Vi-CELL cell counter. ( d ) The levels of cleaved caspase 3, PARP, p-p53-Ser15 and p53 proteins were examined by western blot assays. ( e ) HCT116 p53 +/+ -LIF and its control cells were treated with 5-FU along with or without Stattic. The mRNA levels of p21 and Fas were determined by Taqman real-time PCR and normalized with actin . ( f ) HCT116 p53 +/+ -LIF and its control cells were transfected with siRNA targeting Stat3 (siRNA Stat3-1) or control siRNA, followed by 5-FU treatment. The levels of Stat3, cleaved caspase 3, PARP, p-p53-Ser15 and p53 proteins were determined by western blot assays. Similar results were obtained when a different Stat3 siRNA (siRNA Stat3-2) were used (see Supplementary Fig. 7a ). ( g ) The upregulation of MDM2 by LIF was largely abolished by Stattic. HCT116 p53 +/+ -LIF, RKO p53 +/+ -LIF and their control cells were treated with Stattic. The MDM2 mRNA levels were determined by Taqman real-time PCR and normalized with actin (left panel). The levels of phosphorylated Stat3 at Tyrosine 705 (p-Stat3-Tyr705), Stat3 and MDM2 proteins were examined by western blot assays (right panels). ( h ) Stat3 increased the expression levels of MDM2. The MDM2 mRNA and protein levels were examined in HCT116 p53 +/+ and RKO p53 +/+ cells transfected with Stat3 expression vectors or control vectors. ( i ) Ectopic Stat3 expression reduced the activation and accumulation of p53 protein in response to 5-FU in HCT116 p53 +/+ cells. For a , c , e , g , h , data are presented as mean±s.d. ( n =3). * P <0.001 (Student’s t -test). Full size image Stat3 upregulates ID1 to mediate the effect of LIF on p53 Stat3 is a transcription factor. Upon activation, Stat3 protein forms dimers that translocate to the nucleus to transcriptionally induce their target genes. ID1, the HLH protein inhibitor of differentiation and DNA binding, has been previously reported to upregulate MDM2 in human oesophageal squamous cells [30] . Interestingly, we found that ectopic LIF expression induced the expression of ID1 at both mRNA and protein levels in HCT116 p53 +/+ and RKO p53 +/+ cells ( Fig. 5a ). The induction of ID1 by LIF is mediated through Stat3; ectopic Stat3 expression induced ID1 at both mRNA and protein levels ( Fig. 5b ), whereas blocking Stat3 by Stattic largely abolished the induction of ID1 by LIF in HCT116 p53 +/+ and RKO p53 +/+ cells ( Fig. 5c for HCT116 p53 +/+ cells and Supplementary Fig. 8 for RKO p53 +/+ cells). The induction of ID1 and MDM2 by ectopic LIF expression was also observed in HCT116 p53 −/− and RKO p53 −/− cells, suggesting that the induction of ID1 by LIF is p53 independent ( Supplementary Fig. 9 ). 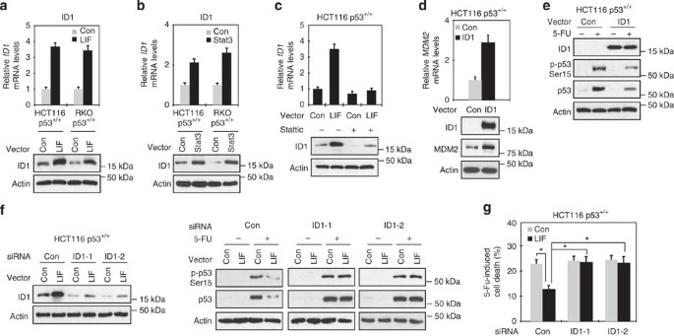Figure 5: Stat3 induces the expression of ID1 to mediate the inhibitory effect of LIF on p53. (a) LIF induced ID1 expression in cultured cells. The mRNA and protein levels of ID1 were determined in HCT116 p53+/+-LIF, RKO p53+/+-LIF and their control cells. (b) Stat3 induced ID1 expression in cultured cells. The mRNA and protein levels of ID1 were determined in HCT116 p53+/+and RKO p53+/+cells transfected with Stat3 expression vectors or control vectors. (c) The induction of ID1 by LIF was largely blocked by Stattic. HCT116 p53+/+-LIF and their control cells were treated with 2 μM Stattic. The expression levels of ID1 were determined at both mRNA and protein levels. (d) Ectopic ID1 expression by expression plasmid (pCMV-ID1) induced MDM2 expression as determined at both mRNA and protein levels in HCT116 p53+/+cells. (e) Ectopic ID1 expression decreased the activation and accumulation of p53 protein in response to 5-FU in HCT116 p53+/+cells. (f) Knockdown of endogenous ID1 by siRNA largely abolished the inhibitory effect of LIF on p53 activation and accumulation in response to 5-FU in HCT116 p53+/+cells. The knockdown of ID1 was confirmed at the protein level (left panel). (g) Knockdown of ID1 largely abolished the inhibitory effect of LIF on 5-FU-induced cell death in HCT116 p53+/+cells. Fora–d,g) data are presented as mean±s.d. (n=3). *P<0.001 (Student’st-test). Figure 5: Stat3 induces the expression of ID1 to mediate the inhibitory effect of LIF on p53. ( a ) LIF induced ID1 expression in cultured cells. The mRNA and protein levels of ID1 were determined in HCT116 p53 +/+ -LIF, RKO p53 +/+ -LIF and their control cells. ( b ) Stat3 induced ID1 expression in cultured cells. The mRNA and protein levels of ID1 were determined in HCT116 p53 +/+ and RKO p53 +/+ cells transfected with Stat3 expression vectors or control vectors. ( c ) The induction of ID1 by LIF was largely blocked by Stattic. HCT116 p53 +/+ -LIF and their control cells were treated with 2 μM Stattic. The expression levels of ID1 were determined at both mRNA and protein levels. ( d ) Ectopic ID1 expression by expression plasmid (pCMV-ID1) induced MDM2 expression as determined at both mRNA and protein levels in HCT116 p53 +/+ cells. ( e ) Ectopic ID1 expression decreased the activation and accumulation of p53 protein in response to 5-FU in HCT116 p53 +/+ cells. ( f ) Knockdown of endogenous ID1 by siRNA largely abolished the inhibitory effect of LIF on p53 activation and accumulation in response to 5-FU in HCT116 p53 +/+ cells. The knockdown of ID1 was confirmed at the protein level (left panel). ( g ) Knockdown of ID1 largely abolished the inhibitory effect of LIF on 5-FU-induced cell death in HCT116 p53 +/+ cells. For a – d , g ) data are presented as mean±s.d. ( n =3). * P <0.001 (Student’s t -test). Full size image To investigate whether ID1 mediates the inhibitory effect of LIF on p53, the effect of ID1 on p53 was determined in HCT116 p53 +/+ cells. Ectopic ID1 expression clearly induced MDM2 at both mRNA and protein levels in HCT116 p53 +/+ cells ( Fig. 5d ), which is similar to the observation in cells with ectopic expression of LIF or Stat3. Furthermore, ectopic ID1 expression reduced the activation and accumulation of p53 protein levels in response to 5-FU treatment ( Fig. 5e ). Importantly, knockdown of endogenous ID1 expression in HCT116 p53 +/+ cells largely reduced the inhibitory effect of LIF on p53 protein levels and 5-FU-induced cell death ( Fig. 5f,g ). These data strongly suggest that Stat3 induces the expression of ID1 to mediate the inhibitory effect of LIF on p53 and p53-mediated apoptosis. LIF promotes chemoresistance in colorectal xenograft tumours To investigate whether the downregulation of p53 by LIF promotes chemoresistance in vivo , the effect of LIF on the therapeutic response to 5-FU was determined in colorectal xenograft tumours. BALB/c nude mice were inoculated with HCT116 p53 +/+ -LIF, HCT116 p53 −/− -LIF and their control cells. When tumours reached the size of ~200 mm 3 , mice were treated with 5-FU (i.p., 30 mg kg −1 daily) for 12 days. 5-FU inhibited the growth of xenograft tumours in a largely p53-dependent manner; 5-FU clearly inhibited the growth of HCT116 p53 +/+ tumours and had much less pronounced effect on HCT116 p53 −/− tumours ( Fig. 6a ). In response to 5-FU treatment, average HCT116 p53 +/+ -Con tumour sizes reduced by 3.2-fold, whereas average HCT116 p53 +/+ -LIF tumour sizes only reduced by 1.4-fold ( P <0.001, Student’s t -test; Fig. 6a ). Notably, the promoting effect of LIF on the therapeutic resistance to 5-FU was greatly reduced in HCT116 p53 −/− tumours ( Fig. 6a ). 5-FU induced p53-mediated apoptosis in HCT116 tumours; 5-FU treatment clearly increased the levels of cleaved caspase 3 and PARP in HCT116 p53 +/+ tumours, but had a very limited effect in HCT116 p53 −/− tumours. Ectopic LIF expression greatly reduced apoptosis induced by 5-FU in HCT116 p53 +/+ tumours; the levels of cleaved caspase 3 and PARP were much lower in HCT116 p53 +/+ -LIF tumours compared with HCT16 p53 +/+ -Con tumours in response to 5-FU treatment ( Fig. 6b ). In contrast, LIF displayed a very limited effect on 5-FU-induced apoptosis in HCT116 p53 −/− tumours ( Fig. 6b ). These results were confirmed by IHC staining of cleaved caspase 3 in HCT116 xenograft tumours; the number of apoptotic cells with positive staining of cleaved caspase 3 were much lower in HCT116 p53 +/+ -LIF tumours compared with HCT116 p53 +/+ -Con tumours ( Fig. 6c ). Consistent with the observation made in in vitro cultured cells, the levels of basal p53 protein and the accumulation of p53 protein in response to 5-FU treatment were much lower in HCT116 p53 +/+ -LIF tumours than HCT116 p53 +/+ -Con tumours ( Fig. 6d ). Furthermore, LIF overexpression activated Stat3, and increased the protein levels of ID1 and MDM2 in HCT116 p53 +/+ xenograft tumours ( Fig. 6e ). These results suggest that the downregulation of p53 protein levels and function is an important mechanism by which LIF promotes chemoresistance in colorectal xenograft tumours. 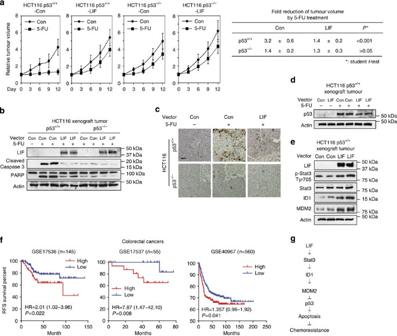Figure 6: LIF promotes chemoresistance in colorectal HCT116 xenograft tumours. (a) LIF promoted chemoresistance towards 5-FU in a largely p53-dependent manner in HCT116 xenograft tumours. HCT116 p53+/+-LIF, HCT116 p53−/−-LIF and their control cells were employed for xenograft tumour formation in nude mice. When tumour volumes reached 200 mm3, mice were treated with 5-FU (30 mg kg−1daily) or vehicle for 12 days. Relative tumour volumes are presented as mean±s.d.,n=8 per group. The fold reduction of tumour volumes by 5-FU was much lower in HCT116 p53+/+-LIF tumours than HCT116 p53+/+-Con tumours, and no clear difference was observed between HCT116 p53−/−-LIF and HCT116 p53−/−-Con tumours.P-value was obtained by analysis of variance, followed by Student’st-tests. (b,c) LIF inhibited 5-FU-induced apoptosis in a largely p53-dependent manner in HCT116 xenograft tumours. (b) The levels of LIF, cleaved caspase 3 and PARP were examined by western blot assays in xenograft tumours. (c) 5-FU-induced apoptosis was determined by IHC staining of cleaved caspase 3 in xenograft tumours. Scale bar, 50 μm. (d). The levels of p53 protein were determined in HCT116 p53+/+-LIF and HCT116 p53+/+-Con tumours treated with and without 5-FU. (e) LIF activated the Stat3 signalling, increased ID1 and MDM2 protein levels in HCT116 p53+/+xenograft tumours. The levels of LIF, total and phosphorylated Stat3 (p-Stat3-Tyr705), ID1 and MDM2 proteins in xenograft tumours formed by HCT116 p53+/+-LIF and HCT1116 p53+/+-Con cells were examined by western blot assays. (f) The correlation between higherLIFlevels and a poor prognosis in relapse-free survival (RFS) of CRC patients. Kaplan–Meier curves indicate the RFS of CRC patients with different expression levels ofLIFfrom three publically available data sets (GSE17536, GSE17537 and GSE40967). The patients whose tumours had higherLIFmRNA levels had significantly shorter RFS than patients whose tumours had lowerLIFmRNA levels.P-value was obtained by Kaplan–Meier statistics and log-rank (one-tail) test. (g) Schematic model depicting the negative regulation of p53 by LIF as an important mechanism that contributes to chemoresistance in human CRCs. Figure 6: LIF promotes chemoresistance in colorectal HCT116 xenograft tumours. ( a ) LIF promoted chemoresistance towards 5-FU in a largely p53-dependent manner in HCT116 xenograft tumours. HCT116 p53 +/+ -LIF, HCT116 p53 −/− -LIF and their control cells were employed for xenograft tumour formation in nude mice. When tumour volumes reached 200 mm 3 , mice were treated with 5-FU (30 mg kg −1 daily) or vehicle for 12 days. Relative tumour volumes are presented as mean±s.d., n =8 per group. The fold reduction of tumour volumes by 5-FU was much lower in HCT116 p53 +/+ -LIF tumours than HCT116 p53 +/+ -Con tumours, and no clear difference was observed between HCT116 p53 −/− -LIF and HCT116 p53 −/− -Con tumours. P- value was obtained by analysis of variance, followed by Student’s t -tests. ( b , c ) LIF inhibited 5-FU-induced apoptosis in a largely p53-dependent manner in HCT116 xenograft tumours. ( b ) The levels of LIF, cleaved caspase 3 and PARP were examined by western blot assays in xenograft tumours. ( c ) 5-FU-induced apoptosis was determined by IHC staining of cleaved caspase 3 in xenograft tumours. Scale bar, 50 μm. ( d ). The levels of p53 protein were determined in HCT116 p53 +/+ -LIF and HCT116 p53 +/+ -Con tumours treated with and without 5-FU. ( e ) LIF activated the Stat3 signalling, increased ID1 and MDM2 protein levels in HCT116 p53 +/+ xenograft tumours. The levels of LIF, total and phosphorylated Stat3 (p-Stat3-Tyr705), ID1 and MDM2 proteins in xenograft tumours formed by HCT116 p53 +/+ -LIF and HCT1116 p53 +/+ -Con cells were examined by western blot assays. ( f ) The correlation between higher LIF levels and a poor prognosis in relapse-free survival (RFS) of CRC patients. Kaplan–Meier curves indicate the RFS of CRC patients with different expression levels of LIF from three publically available data sets (GSE17536, GSE17537 and GSE40967). The patients whose tumours had higher LIF mRNA levels had significantly shorter RFS than patients whose tumours had lower LIF mRNA levels. P- value was obtained by Kaplan–Meier statistics and log-rank (one-tail) test. ( g ) Schematic model depicting the negative regulation of p53 by LIF as an important mechanism that contributes to chemoresistance in human CRCs. Full size image LIF is associated with a poor prognosis in CRC patients To further evaluate the clinical importance of LIF in CRC, the prognostic value of LIF mRNA expression was analysed in three publically available data sets of CRC patients (GSE17536, GSE17537 and GSE40967). Patients were divided into two groups according to the mean expression levels of LIF mRNA. As shown in Fig. 6f , there was a significant association of high LIF expression levels with a poor prognosis of relapse-free survival in all three cohorts tested. These results suggest that high LIF levels predict a poor prognosis of CRC patients, which supports our results from both cultured cells and mouse tumour models. Taken together, these results clearly demonstrated that LIF attenuates p53 function, which in turn promotes the therapeutic resistance to 5-FU, and could be a prognostic marker for poor relapse-free survival in CRC patients. LIF is a multifunctional cytokine that plays a wide array of functions depending on cell and tissue types. LIF is essential for the maintenance of mouse embryonic stem cell pluripotency, regulation of inflammation and also plays a critical role in blastocyst implantation [19] , [21] , [31] . Our recent studies demonstrated that LIF is a p53 target and mediates p53 function in reproduction [25] , [27] , [28] . LIF expression in uterus is under the control of p53, especially at the implantation stage, to ensure the proper embryonic implantation. Loss of p53 in female mice leads to impaired implantation [25] . The deceased activity of the p53 pathway is associated with the decreased maternal fertility in human populations [27] . Although LIF functions as a downstream target of p53 to mediate p53 function in maternal reproduction, results from this study clearly demonstrated an additional important role of LIF in regulating p53 levels and function in tumour suppression in CRCs. LIF downregulates p53 protein levels and function, including transcriptional activity, apoptosis and senescence, which forms a negative feedback loop with p53. Results in this study further showed that LIF is overexpressed in a large percentage of human CRCs and is associated with a poor prognosis of CRC patients. Overexpression of LIF promotes chemoresistance in cultured CRC cells and colorectal xenograft tumours in a largely p53-dependent manner ( Fig. 6g ). Therefore, overexpression of LIF could be an important factor contributing to the chemoresistance in CRCs. The pleiotropic effects of LIF signalling is mainly due to the selective activation of different kinases, including JAKs, MAPK, PI3K, and transcription factors, including Stat3, AP1, in a highly context-dependent manner. In this study, we investigated the mechanisms by which LIF negatively regulates p53. We found that the inhibitory effect of LIF on p53 is largely mediated by the activation of Stat3. Blocking the Stat3 pathway largely abolishes the inhibitory effect of LIF on p53. Stat3 is frequently activated in many types of human cancers, including CRC, and is crucial to the survival and growth of tumour cells [32] , [33] , [34] , [35] . The regulation of mouse p53 by Stat3 has been suggested by a previous study showing that Stat3 binds to the promoter of mouse p53 gene and inhibits p53 expression at the mRNA level in mouse cell lines [36] . In this study, we found that Stat3 downregulates p53 protein levels but has no apparent effect on p53 mRNA levels in human cells. Furthermore, we found that Stat3 can upregulate MDM2, a key negative regulator of p53 protein, which is an unidentified mechanism by which Stat3 downregulates p53 in human CRC. Together, these findings suggest that Stat3 negatively regulates p53 in both mouse and human cell lines, but through different mechanisms. We further identified that Stat3 transcriptionally induces ID1 to mediate its role in the negative regulation of p53. ID1 is often under the transcriptional regulation by the bone morphogenetic proteins (BMPs)/Smad pathway. BMP activates Smad1/5, which binds to Smad4, then translocates to the nucleus and binds to Smad-binding elements in the promoter of ID1 to induce ID1 transcription [37] , [38] . In addition to the BMP/Smad pathway, ID1 can also be transcriptionally regulated by Scr, early growth response protein 1 (refs 39 , 40 ). Results in this study demonstrated that Stat3 is an additional important regulator of ID1 expression. Consistently, analysis of a panel of supratentorial primitive neuroectodermal tumours showed the activation of the Stat3 pathway along with the increased mRNA expression of ID1 , suggesting the possible regulation of ID1 by the Stat3 pathway in primitive neuroectodermal tumours [41] . ID1 belongs to a family of HLH transcriptional regulatory factors, which is involved in the regulation of gene expression. ID1 often functions as a transcription repressor through heterodimerization with the basic HLH transcription factors to inhibit their transcriptional function [42] . ID1 has also been shown to upregulate the expression of some genes through different mechanisms [43] , [44] , [45] , [46] . For example, ID1 has been shown to induce VEGF transcription by stabilizing hypoxia-inducible factor 1α protein [43] . ID1 can activate nuclear factor κB signalling and upregulate its target genes, including Bcl-xL and ICAM-1 (ref. 45 ). It has also been reported that ID1 upregulates MMP-2 and EGF-R [44] , [46] . ID1 plays an important role in development, stem cell self-renewal activity, senescence, differentiation, angiogenesis and migration [47] . Overexpression of ID1 has been reported in a variety of human cancers, including CRC, and is often associated with poor prognosis and chemoresistance [48] , [49] , [50] , [51] . In this study, we found that overexpression of ID1 clearly increases MDM2 mRNA and protein levels in human CRC cells, which in turn downregulates p53 protein levels. Currently, it is still unclear how ID1 transcriptionally regulates MDM2 , which needs further studies in the future. Importantly, knockdown of endogenous ID1 largely abolishes the effect of LIF on MDM2 and p53, demonstrating that downregulation of p53 by the LIF/Stat3 signalling is largely mediated by ID1 ( Fig. 6g ). The role of LIF in cancer and its underlying mechanisms are not well understood. LIF has been shown to have a complex role in cancer from limited studies. LIF can induce the differentiation of murine myeloid leukaemia cells and suppress their proliferation [52] . Meanwhile, LIF displays a promoting effect on tumorigeneis in many solid tumours [53] , [54] , [55] . LIF promotes proliferation of cancer cell lines, and is involved in the metastasis of cells from breast cancer, rhabdomyosarcoma, melanoma and nasopharyngeal carcinoma [54] , [55] , [56] , [57] . The increased expression levels of LIF are associated with poor prognosis in patients of breast cancer and nasopharyngeal cancer [54] , [55] . Results in this study showed that LIF promotes chemoresistance towards a group of chemotherapeutic agents in CRC, and demonstrated that the downregulation of p53 by LIF is an important underlying mechanism. However, majority of these results were obtained by using engineered cell lines with ectopic LIF expression or knockdown of endogenous LIF. Considering the limitation of engineered cell lines, it will be important to confirm the effect of LIF on chemoresistance and its underlying mechanisms in primary human tumours in future studies. Clinical studies show that ~50% of CRC patients develop recurrent disease despite the use of surgical resection and chemotherapy. By employing several publically available data sets of CRC patients, we found that high LIF levels in tumours are associated with shorter recurrent-free survival of CRC patients. In summary, this study demonstrates that LIF, which is overexpressed in a large percentage of human CRCs, is an important negative regulator of p53 through activating the Stat3/ID1/MDM2 pathway, which in turn promotes chemoresistance in CRC. Targeting LIF, Stat3 as well as ID1 to reactivate p53 is a potential therapeutic strategy to enhance chemosensitivity in CRC, especially in tumours with LIF overexpression. Cell culture and cell treatments Human CRC HCT116 p53 +/+ , HCT116 p53 −/− , RKO p53 +/+ , RKO p53 −/− , DLD-1 p53 +/+ and DLD-1 p53 −/− cell lines were generous gifts from Dr Bert Vogelstein, Johns Hopkins University. Cells with stable ectopic LIF expression were established by transduction of a retroviral LIF expression vector (pLPCX-LIF) and selected by puromycin. Cells with inducible p53 expression (H1299-Tet-on-p53) were established by stable transfection of a Tet-on p53 expression vector (Life Technology) into p53-null human H1299 cells, which express p53 only in the presence of doxycycline. CM was collected after serum-free medium was cultured overnight with cells. Human Stat3 expression vector (EF.STAT3C.Ubc.GFP vector) was constructed by the group of Dr L. Resar at Johns Hopkins University [58] . pCMV-ID1 expression vector was constructed by amplifying ID1 cDNA using following primers: forward: 5′-CCCAAGCTTATGAAAGTCGCCAGTGGCA-3′; reverse: 5′-CGGGATCCGCGACACAAGATGCGATCGT-3′, and inserting ID1 fragment into p3XFlag-CMV-14 vectors (Sigma). Expression plasmids were transfected into cells using Lipofectamine 2000 (Invitrogen). For siRNA knockdown, two different siRNA oligos against LIF , Stat3 and ID1 , respectively, were purchased from IDT. siRNA target LIF : siRNA-1: 5′-CAACAACCUGGACAAGCUAUGUGGC-3′; siRNA-2: 5′-GUCACAACCUCAUGAACCAGAT-3′. siRNA target Stat3 : siRNA-1: 5′-UCCAGUUUCUUAAUUUGUUGACGGGUC-3′; siRNA-2: 5′-AUAGUCCUAUCUUCUAUUUGGAUGUCA-3′. siRNA target ID1 : siRNA-1: 5′-AUAUUACAAUGAUCACCGACUGAAA-3′; siRNA-2: 5′-GGAAUUACGUGCUCUGUGGGUCUCC-3′. Two different siRNA oligos against MDM2 were purchased from Qiagen (Cat#SI00300846) and Dharmacon (Cat#M-003279-01). 5-FU, ETO, ADR, MG132, cycloheximide, Doxorubicin and Stattic were purchased from Sigma. Tissue samples The Colon Cancer cDNA array that contains 24 pairs of cDNA prepared from human CRC samples and their matched adjacent non-tumour tissues was purchased from Origene. Twenty-five cases of formalin-fixed and paraffin-embedded primary CRC samples and their matched adjacent non-tumour tissues were collected at the University of Texas MD Anderson Cancer Center with approval from institutional review board. Western blot assays Standard western blot assays were used to analyse the levels of protein in cell lysates and CM. CM that was cultured with one-third number of the cells used for western blot assays was concentrated with an Amico Ultra-4 centrifugal filter device (Millipore) after a brief centrifugation to remove any cell debris. Antibodies against p53 (FL393, Santa Cruz; 1:1,000 dilution), anti-p-p53 (Ser15) (9284, Cell Signaling; 1:1,000 dilution), anti-LIF (AF-250-NA, R&D; 1:1,000 dilution), anti-PARP1/2 (H250, Santa Cruz; 1:1,000 dilution), anti-cleaved-caspase 3 (D175, Cell Signaling; 1:1,000 dilution), anti-MDM2 (2A10; 1:1,000 dilution), anti-p-Stat3 (Tyr705) (9131, Cell Signaling; 1:1,000 dilution), anti-Stat3 (C-20, Santa Cruz; 1:2,000 dilution), anti-ID1 (C-20, Santa Cruz; 1:2,000 dilution), anti-p21 (Ab-6, Calbiochem; 1:1,000 dilution) and anti-β-actin (A5441, Sigma; 1:125,000 dilution) antibodies were used in this study. The full blots are shown in Supplementary Figs 10 – 14 . IF staining assays IF staining was performed as previously described [59] . In brief, cells grown on slides were fixed with 4% paraformaldehyde for 30 min and treated with 0.5% Triton X-100 for 5 min, blocked with 1% bovine serum albumin for 30 min, and stained with anti-p53 (FL393; 1:300 dilution) and anti-Flag (1:200 dilution) antibodies overnight at 4 °C to detect p53 and LIF-Flag, respectively. Slides were washed and then incubated with Alexa Fluor 555 Goat Anti-Mouse IgG (H+L) (Invitrogen) and Alexa Fluor 488 Goat Anti-Rabbit IgG (H+L) (Invitrogen). Nuclei were stained with 4′,6-diamidino-2-phenylindole (Vector). Taqman real-time PCR Total RNA was prepared by using an RNeasy kit (Qiagen). All primers were purchased from Applied Biosystems. Real-time PCR was done in triplicate with TaqMan PCR mixture (Applied Biosystems). The expression of genes was normalized to the actin gene. Assays for cell viability and Annexin V staining The Vi-CELL cell counter (Beckman Coulter) that performs a trypan blue exclusion method was employed to determine cell viability. Apoptosis was measured by staining cells using Muse Annexin V & Dead Cell Assay Kit (Millipore) and analysing cells in the Muse Cell Analyzer (Millipore), which is a bench flow cytometry, according to the manufacturer’s instructions. Cell sorting HCT116 p53 +/+ -LIF and their control cells treated with 5-FU were trypsinized, washed with PBS and stained with Alexa Fluor 488 Annexin V according to the manufacturer’s protocol (Invitrogen). After staining, cells were analysed and cells negative for Annexin V staining were sorted by a BD Biosciences ultra-high-speed Influx cell sorter (BD Biosciences). Cellular senescence analysis Cells were treated with doxorubicin (50 nM) for 3 days. Senescent cells were detected by senescence-associated β-galactosidase assays using a Senescence β-Galactosidase Staining Kit (Cell Signaling). 5-FU treatment of colorectal xenograft tumours The 7-week-old BALB/c nu/nu male athymic nude mice (Taconic) were inoculated (via s.c. injection) with HCT116 p53 +/+ and HCT116 p53 −/− cells with or without ectopic LIF expression (5 × 10 6 in 0.2 ml PBS) for xenograft tumour formation. When tumour volumes reached 200 mm 3 , mice were treated with 5-FU (i.p., 30 mg kg −1 daily) or vehicle for 12 days. Tumour volume and mouse weight were monitored three times per week. The mouse experiments were performed with the approval of the Institutional Animal Care and Use Committee of Rutgers State University of New Jersey. IHC staining assays IHC staining for LIF and Cleaved-caspase 3 was performed as previously described [60] . In brief, tissue sections were deparaffinized in xylene and rehydrated with ethanol. After pre-incubation with 10% normal goat serum in PBS (pH 7.5), tissue sections were incubated with primary antibodies, including anti-LIF (AF-250-NA, R&D, 1:100 dilution) and anti-Cleaved caspase 3 antibodies (D175, Cell Signaling, 1:1,000 dilution), for overnight at 4 °C. Tissue sections were then stained with biotinylated secondary antibody (Vector). Immunoreactivity was detected by using a Vectastain Elite ABC kit (Vector). Known positive controls were included in each experiment, and negative controls were obtained by omitting the primary antibody. The IHC results were scored according to the percentage of cells showing positive staining: −: 0% to <10%; +: ≥10%. Data sets of CRC patients Three cohorts of CRC patients with known LIF mRNA expression levels and relapse-free survival information were obtained from publically available data sets (GSE17536, GSE17537 and GSE40967) [61] , [62] , [63] . Genome-wide expression levels of all tumour specimens were assessed on Affymetrix HGU133 Plus 2.0 arrays (Affymetrix). To analyse the prognostic value of LIF expression levels, the patients were split into two groups according to the mean expression levels of LIF in tumours. Statistical analysis The data were expressed as mean±s.d. The differences in xenograft tumour size in response to 5-FU treatment were analysed for statistical significance by analysis of variance, followed by Student’s t -tests using a GraphPad Prism software. Kaplan–Meier statistics and log-rank (one-tail) test were performed to estimate the significance of differences in relapse-free survival of patients among different groups. All other P -values were obtained using two-tailed Student’s t -tests. The results were considered to be significant, when P value<0.05. How to cite this article: Yu, H. et al. LIF negatively regulates tumour-suppressor p53 through Stat3/ID1/MDM2 in colorectal cancers. Nat. Commun. 5:5218 doi: 10.1038/ncomms6218 (2014).